Protein-binding assays in biological liquids using microscale thermophoresis Protein interactions inside the human body are expected to differ from the situation in vitro . This is crucial when investigating protein functions or developing new drugs. In this study, we present a sample-efficient, free-solution method, termed microscale thermophoresis, that is capable of analysing interactions of proteins or small molecules in biological liquids such as blood serum or cell lysate. The technique is based on the thermophoresis of molecules, which provides information about molecule size, charge and hydration shell. We validated the method using immunologically relevant systems including human interferon gamma and the interaction of calmodulin with calcium. The affinity of the small-molecule inhibitor quercetin to its kinase PKA was determined in buffer and human serum, revealing a 400-fold reduced affinity in serum. This information about the influence of the biological matrix may allow to make more reliable conclusions on protein functionality, and may facilitate more efficient drug development. Methods to analyse proteins and their interactions with other biomolecules or low-molecular-weight compounds are of great importance for the evaluation of cellular functions and for the development of pharmaceuticals. Potential drug candidates range from specifically designed antibodies to low-molecular-weight compounds that inhibit or activate cellular processes. Although there is a variety of in vitro approaches that can address particular interactions, there is a constant need for new techniques. In particular, the analysis of binding processes of small molecules and the general complications of making measurements in biological liquids remain significant challenges in modern bioanalytics. Recent technological advances have indicated that thermophoresis could provide the means for such interaction analyses. Thermophoresis is the directed motion of molecules induced by temperature gradients. It was first discovered by Ludwig [1] and since then has been a subject of research mostly using inorganic molecules or polymer blends [2] , [3] . Braun and Libchaber [4] , as well as Piazza [5] , measured the thermophoresis of biomolecules to understand the intricacies of the effect [6] , [7] , [8] . Recently, Baaske et al . [9] showed that thermophoresis is capable of analysing DNA aptamer interactions with thrombin and ATP. Although these experiments demonstrate that it is possible to quantify interactions using thermophoresis, DNA aptamers are known for a strong thermophoretic effect due to their high charge [10] . Hence, the binding of the large protein thrombin or the highly charged ATP results in a strong thermophoretic response. In this study, we introduce microscale thermophoresis (MST) as a tool to characterize protein and small-molecule interactions in buffers and biological liquids. Such analyses are usually difficult as the thermophoresis of proteins is generally weak. In addition, low-molecular-weight binders often do not significantly change the charge or size of a molecule, but only induce weak conformational changes on binding. Hence, the analysis of potential drug candidates is far more challenging. The results presented in this study, however, demonstrate that MST is highly suitable for these kinds of interaction studies. In contrast to existing techniques, MST works in free-solution and with low consumption of sample. It is an entirely optical method, which is contact-free and therefore minimizes contamination of the sample. A simple Mix&Read protocol renders complex preparations unnecessary. To show the wide applicability of MST, we quantified the dissociation constants of various protein interactions both in buffer and in solutions similar to the protein's native environment, namely, blood serum or cell lysate. Experimental approach The experimental setup consists of an infrared laser coupled into the path of fluorescent excitation/emission using an infrared dichroic mirror ( Fig. 1a ). The laser is focused onto the sample through the same objective that is used for fluorescence detection. This allows the observation of thermohoresis in various microfluidic sample compartments such as capillaries or microfluidic channels. High reproducibility and low sample consumption are achieved using 100-μm-diameter glass capillaries with a total volume of about 500 nl. The infrared-laser creates a spatial temperature distribution on the length scale of 25 μm. The temperature increase scales linearly with the laser power. After 150 ms, laser heating and heat dissipation reach equilibrium, and a steady-state temperature increase of typically 2–6 K is obtained. This temperature rise induces a spatial concentration distribution that is visualized by a fluorescent dye covalently attached to one of the binding partners. Typically, one primary amine per protein is labelled and thus the position of the dye is statistically distributed. Given the number of lysines on a typical protein, the chance that the label interferes with the binding is very low. The majority of proteins are labelled far from the binding site, disturbing the interaction only minimally. To measure thermophoresis of proteins, the change in concentration between the initial state and the steady state is measured. Therefore, two images of the sample are required: one image of the initial state before laser heating, showing a homogenous distribution of molecules, and a second image acquired after a few seconds of infrared-laser heating ( Fig. 1b ). This short measurement time is sufficient because of the fast mass diffusion over the small dimension of the temperature distribution. Even if the diffusion is slow and no steady state is reached within the measurement time, the concentration profiles are typically distinguishable after several seconds. Switching off the infrared-laser leads to a re-establishment of the initial homogeneous concentration profile by ordinary diffusion, providing information about the diffusion coefficient of the molecules [11] . 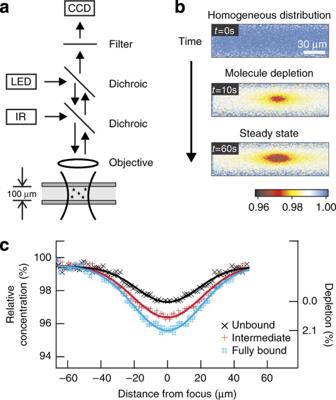Figure 1: Setup and principle of MST. (a) Experimental approach. With an additional dichroic mirror inserted into an epifluorescence microscope, a heating infrared-laser is focused into a fused silica capillary with an inner diameter of 100 μm. The sample fluorescence is imaged with a CCD camera. (b) Fluorescence images. Fluorescence images are acquired over time. Initially, fluorescently labelled molecules are distributed evenly. After switching on the heating with a focused infrared-laser, the molecules experience the thermophoretic force in the temperature gradient and typically move out of the heated spot. In the steady state, this molecule flow is counterbalanced by ordinary mass diffusion and a steady-state concentration profile is established. The colour code indicates the relative fluorescence in the sample. (c) Steady-state profiles. The steady-state profiles of human interferon-γ are plotted for various concentrations of a binding antibody (black ×: 0.1 nM, red plus sign: 80 nM, blue number sign: 500 nM). The depletion directly reflects the fraction of bound complex. Figure 1: Setup and principle of MST. ( a ) Experimental approach. With an additional dichroic mirror inserted into an epifluorescence microscope, a heating infrared-laser is focused into a fused silica capillary with an inner diameter of 100 μm. The sample fluorescence is imaged with a CCD camera. ( b ) Fluorescence images. Fluorescence images are acquired over time. Initially, fluorescently labelled molecules are distributed evenly. After switching on the heating with a focused infrared-laser, the molecules experience the thermophoretic force in the temperature gradient and typically move out of the heated spot. In the steady state, this molecule flow is counterbalanced by ordinary mass diffusion and a steady-state concentration profile is established. The colour code indicates the relative fluorescence in the sample. ( c ) Steady-state profiles. The steady-state profiles of human interferon-γ are plotted for various concentrations of a binding antibody (black ×: 0.1 nM, red plus sign: 80 nM, blue number sign: 500 nM). The depletion directly reflects the fraction of bound complex. Full size image To analyse binding events, the measurement is performed at various concentration ratios of the binding partners. Typically, the fluorescent binding partner is kept at a constant concentration and the unlabelled molecule is titrated until a saturation of all binding sites is obtained. Figure 1c shows the steady-state profiles of human interferon gamma (hIFN-γ) at various concentrations of a specific antibody. At low antibody concentrations, the profile reflects the thermophoresis of the unbound protein, whereas at high concentrations it indicates that of the complex. For intermediate concentrations, the measured depletion is a linear superposition of the bound and unbound states: In Equation (1) Δ c measured is the measured depletion, Δ c bound and Δ c unbound represent depletion of the bound and unbound states, respectively, and f is the fraction of molecules in the bound state. The concentration change in the focal area can be directly transferred into a binding curve when plotted against the concentration of the added binding partner. From these data, the equilibrium dissociation constant K d and a potential cooperativity can be determined. Protein interactions Specific interactions between proteins have a fundamental role in cellular functions and are important for biotechnological applications and antibody-based assays. In the following, we apply MST in several typical experiments to show its feasibility for use in interaction studies in the course of drug development or pharmaceutical research. First, we determined the affinity of an antibody for its antigen analysing the interaction of an anti-IFN-γ antibody (120 kDa) with its antigen, hIFN-γ (17 kDa). hIFN-γ is a dimerized soluble cytokine that is crucial for immunity against intracellular pathogens and also for tumour control [12] . The hIFN-γ was labelled with AlexaFluor 647 and kept at a constant concentration of 5 nM in 1× phosphate-buffered saline (PBS) buffer at 5 °C. The antibody was titrated from 0.1 to 700 nM. On binding of the antibody, the thermophoretic concentration signal of hIFN-γ ranged from 2.14% for the unbound hIFN-γ to 4.24% for the bound complex, resulting in a differential depletion of 2.1% for the binding reaction. 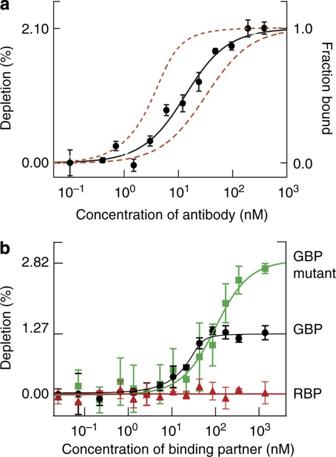Figure 2: Protein–protein interactions measured with MST. To determine the affinity of a binding reaction, a titration series of one binding partner is performed while the fluorescent binding partner is kept at a constant concentration. (a) The binding of fluorescently labelled hIFN-γ to a specific antibody is analysed with MST (black circles). The antibody is titrated from 100 pM to 700 nM. The change in the thermophoretic signal leads to aKd=10±2 nM. For comparison, the dashed lines show binding curves for 1 and 30 nM. (b) The interaction of the intrinsic fluorescent protein GFP with binders of varying affinities is measured. The GBP shows a high affinity of 2.3±2.1 nM (black circles), which is confirmed by a reference experiment on an Attana quartz crystal microbalance device. To ensure that the measured interaction truly represents specific binding, a GBP mutant (R37A) and non-binding RBP are further analysed with MST. The exchange of the arginine at the binding interface reduces the affinity to 80±38 nM (green squares), while the RBP shows the expected baseline (red triangles). The error bars represent the s.d. of each data point calculated from three independent thermophoresis measurements. The level of depletion, as compared with the unbound state, versus the antibody concentration is plotted in Figure 2a . As discussed in the previous section, the depletion can be interpreted as a binding curve with the fraction of hIFN-γ in complex with its antibody plotted on the right axis. Fitting the data according to Equation (4) results in a dissociation constant of K d =10±2 nM. To show the high resolution of MST, we plotted the expected binding behaviour for K d =1 and 30 nM. Figure 2: Protein–protein interactions measured with MST. To determine the affinity of a binding reaction, a titration series of one binding partner is performed while the fluorescent binding partner is kept at a constant concentration. ( a ) The binding of fluorescently labelled hIFN-γ to a specific antibody is analysed with MST (black circles). The antibody is titrated from 100 pM to 700 nM. The change in the thermophoretic signal leads to a K d =10±2 nM. For comparison, the dashed lines show binding curves for 1 and 30 nM. ( b ) The interaction of the intrinsic fluorescent protein GFP with binders of varying affinities is measured. The GBP shows a high affinity of 2.3±2.1 nM (black circles), which is confirmed by a reference experiment on an Attana quartz crystal microbalance device. To ensure that the measured interaction truly represents specific binding, a GBP mutant (R37A) and non-binding RBP are further analysed with MST. The exchange of the arginine at the binding interface reduces the affinity to 80±38 nM (green squares), while the RBP shows the expected baseline (red triangles). The error bars represent the s.d. of each data point calculated from three independent thermophoresis measurements. Full size image We further analysed a recently described interaction between green fluorescent protein (GFP) and a small antibody fragment known as GFP-binding protein (GBP) [13] , which is derived from a single domain antibody of a Llama Alpaca ( Fig. 2b ). It was previously shown that GBP efficiently binds its antigen (GFP) in living cells as well as in immune-precipitation assays [13] . As GFP is intrinsically fluorescent, no fluorescent label was necessary to monitor the interaction. We prepared a titration series with a constant GFP concentration of 40 nM and varying amounts of GBP. The dissociation coefficient was determined to be K d =2.3±2.1 nM, which is 25-fold lower than the concentration of GFP. Still, determination was possible with fair accuracy by accounting for ligand depletion. We directly compared the obtained K d with affinity studies carried out on an Attana surface sensor instrument using a quartz crystal microbalance sensor (QCM). For this experiment, GBP was immobilized on the QCM surface and the on- and off-rates of GFP were determined, resulting in a dissociation constant of 0.63 nM. From a comparison of various interaction techniques, it is known that surface-based methods tend to overestimate the affinity of an interaction [14] . With this in mind, the affinities determined with MST and QCM are in good agreement. To determine whether the measured MST response represents specific binding, we analysed the interaction of a GBP carrying a mutation at its binding site. At position 37, an arginine was replaced by an alanine, which is known to reduce the binding affinity (see Supplementary Information ). Furthermore, a non-binding protein, the red fluorescent protein (RFP)-binding protein (RBP), was analysed to exclude non-specific contributions. We found a binding affinity of 80±38 nM for the GBP mutant and no binding for RBP. Interestingly, the depletion changed from 1.27 to 2.82% for GBP and the GBP mutant (R37A), respectively. This is due to the fact that the thermophoretic amplitude not only depends on the size of the complex but also contains contributions from both charge and structure. By replacing a charged arginine by a structurally different and uncharged alanine, a resulting influence on the complex is very likely and can be observed in the thermophoretic amplitude. Low-molecular-weight binding The high sensitivity of thermophoresis for the binding of low-molecular-weight ligands is demonstrated by measuring the interaction of calmodulin (CaM, 16.7 kDa) with Ca 2+ ions ( Fig. 3a ). CaM is the primary receptor for calcium ions in human cells, acting as a mediator of calcium functions and regulating many cellular processes [15] . Depending on its conformational state, CaM binds or regulates a multitude of protein targets. On binding to calcium, CaM undergoes a conformational change, rearranging more than 35 water molecules per CaM [16] , which leads to a significant change in the thermophoretic properties. For analysing the binding behaviour, we performed a titration series from 1 nM to 50 μM Ca 2+ ions, with 150 nM CaM kept constant throughout the series. We infer a dissociation constant of 2.8±0.2 μM and a cooperativity of 1.97±0.2. This value is in good agreement with the reported K d values for CaM–Ca 2+ in the affinity range from 1 to 10 μM [17] . As a control for specificity of the thermophoretic signal, a similar experiment was performed with Mg 2+ ions instead of Ca 2+ ions. Both ion species are equal in charge and similar in size. As no change in depletion was observed as a function of changing Mg 2+ concentration, non-specific binding was excluded and the specificity of calcium ion binding to CaM was confirmed. 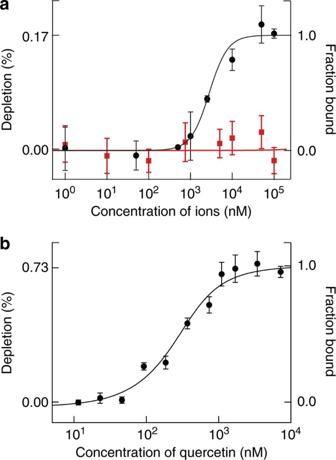Figure 3: Analysis of the binding of ions and small molecules. (a) Binding of Ca2+ions to fluorescently labelled CaM is quantified in PBS buffer. The concentration of calcium ions was varied from 1 nM to 100 μM, while the concentration of the protein CaM was kept constant at 150 nM. To test for specificity of the interaction, the same titration series was performed with magnesium ions. For Ca2+, we found a dissociation constant ofKd=2.8±0.2 μM (black circles), whereas no binding was observed for Mg2+ions (red squares). (b) The binding of the small, uncharged inhibitor quercetin to the cAMP-dependent kinase PKA is measured with MST (black circles). The titration of quercetin ranged from 11.5 nM to 50 μM with a constant concentration of the labelled kinase at 300 nM. Despite the small changes in the molecule's mass, a signal-to-noise ratio of 12.5 allows an accurate determination of the interaction strength. The affinity is determined to be 130±30 nM, in good agreement with reported values. The error bars represent the s.d. of each data point calculated from three independent thermophoresis measurements. Figure 3: Analysis of the binding of ions and small molecules. ( a ) Binding of Ca 2+ ions to fluorescently labelled CaM is quantified in PBS buffer. The concentration of calcium ions was varied from 1 nM to 100 μM, while the concentration of the protein CaM was kept constant at 150 nM. To test for specificity of the interaction, the same titration series was performed with magnesium ions. For Ca 2+ , we found a dissociation constant of K d =2.8±0.2 μM (black circles), whereas no binding was observed for Mg 2+ ions (red squares). ( b ) The binding of the small, uncharged inhibitor quercetin to the cAMP-dependent kinase PKA is measured with MST (black circles). The titration of quercetin ranged from 11.5 nM to 50 μM with a constant concentration of the labelled kinase at 300 nM. Despite the small changes in the molecule's mass, a signal-to-noise ratio of 12.5 allows an accurate determination of the interaction strength. The affinity is determined to be 130±30 nM, in good agreement with reported values. The error bars represent the s.d. of each data point calculated from three independent thermophoresis measurements. Full size image The binding of an uncharged low-molecular-weight inhibitor to its target can also be analysed with MST. The cAMP-dependent kinase (PKA, 38 kDa) was analysed against the inhibitor quercetin (0.34 kDa; Fig. 3b ). The kinase was fluorescently labelled and kept at a concentration of 300 nM. The inhibitor quercetin was titrated up to 50 μM in 50 mM HEPES buffer and 5% dimethyl sulphoxide (DMSO). We found an affinity of 130±35 nM, which is in good agreement with the literature, where affinities of quercetin for various kinases are reported in the nanomolar to micromolar range [18] , [19] . In this experiment, the thermophoretic concentration signal changed from 3.8% for the unbound state to 4.53% for the bound state, showing a 19% relative change on binding of quercetin. As the mass of the bound complex differed by only 1% and charge contributions are unlikely, we attribute the large signal to changes in the hydration shell originating from water molecules that are either displaced from the binding pocket or reorganized when the protein undergoes conformational changes. The experiments presented in this study demonstrate that MST is suitable for the analysis of low-molecular-weight binders. Owing to the high precision when analysing the thermophoretic signal, ion binding is still detectable with a signal-to-noise ratio of 5. In the case of quercetin binding, a signal-to-noise ratio of 12.5 was achieved, demonstrating that even minor changes are detectable with MST. Competitive binding in cell lysate and serum Today, analyses of protein interactions are typically performed in buffered salt solutions, which mimic natural conditions. However, these solutions lack many components that are present in the original biological liquid and that can have significant effects on the binding behaviour. An analysis in these artificial systems cannot provide precise information about the binding behaviour inside the human body and may lead to wrong decisions when developing drug candidates. As shown below, MST can analyse interactions of proteins and small molecules in complex biological liquids, gathering information on binding under conditions close to the in vivo situation. By using a red-fluorescent label, we avoided background fluorescence caused by the intrinsic fluorescence of proteins in crude cell extract or blood serum. We found that, in cell extracts, binding was dramatically shifted to lower affinities ( Fig. 4a ). For hIFN-γ, the apparent dissociation constant was determined to be 165±26 nM in the cell extract, compared with 10±2 nM in PBS buffer. Affinities of biomolecules seem to be highly dependent on the composition of the surrounding matrix. Such significant affinity reduction might be caused by competitive interactions with components of the biological liquid or could also be due to differences in viscosity, pH or ionic strength [9] . Using only microliter volumes, MST might be able to measure the affinity of unpurified, expressed antibodies directly in the supernatant of a cell suspension, opening novel ways for fast antibody selection. 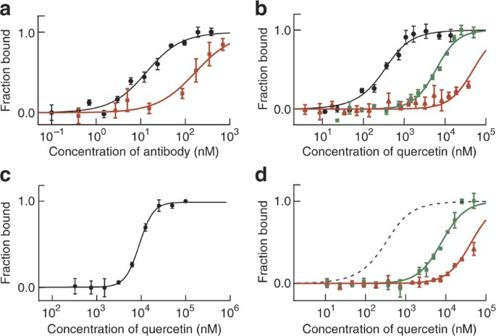Figure 4: Thermophoretic analysis of interactions in biological liquids. (a) The interaction of hIFN-γ with a specific antibody is analysed in buffer and compared with the same interaction in crudeE.colicell lysate. The affinity is shifted from 10±2 nM in buffer (black circles) to 165±26 nM in cell lysate (red squares). (b) The binding of the inhibitor quercetin to the cAMP-dependent kinase PKA is analysed in human serum. There, the apparent dissociation constantKdchanges from 0.13±0.04 μM (black circles) to 6±0.4 μM in 5% human serum (green squares) and to 50±7 μM in 30% human serum (red triangles). (c) The binding of quercetin to the blood protein HSA is quantified using MST (black circles). The data yield a dissociation constantKd=9.3±0.5 μM and a cooperativity of 2.75±0.2. (d) When using HSA concentrations corresponding to 5 and 30% human serum, a result comparable to the situation in real human serum was obtained. At a concentration of 32 μM HSA, the apparent affinity shifted toKd=7.8±0.6 μM (green squares), while at 190 μMHSA Kd=43±6 μM (red triangles). The black dashed line represents the binding of quercetin to PKA in buffer. The error bars represent the s.d. of each data point calculated from three independent thermophoresis measurements. Figure 4: Thermophoretic analysis of interactions in biological liquids. ( a ) The interaction of hIFN-γ with a specific antibody is analysed in buffer and compared with the same interaction in crude E . coli cell lysate. The affinity is shifted from 10±2 nM in buffer (black circles) to 165±26 nM in cell lysate (red squares). ( b ) The binding of the inhibitor quercetin to the cAMP-dependent kinase PKA is analysed in human serum. There, the apparent dissociation constant K d changes from 0.13±0.04 μM (black circles) to 6±0.4 μM in 5% human serum (green squares) and to 50±7 μM in 30% human serum (red triangles). ( c ) The binding of quercetin to the blood protein HSA is quantified using MST (black circles). The data yield a dissociation constant K d =9.3±0.5 μM and a cooperativity of 2.75±0.2. ( d ) When using HSA concentrations corresponding to 5 and 30% human serum, a result comparable to the situation in real human serum was obtained. At a concentration of 32 μM HSA, the apparent affinity shifted to K d =7.8±0.6 μM (green squares), while at 190 μM HSA K d =43±6 μM (red triangles). The black dashed line represents the binding of quercetin to PKA in buffer. The error bars represent the s.d. of each data point calculated from three independent thermophoresis measurements. Full size image Low-molecular-weight binders such as those discussed in the previous section are often likely candidates for new drugs. With MST, small-molecule interactions can also be quantified in complex biological liquids. We performed the quercetin titration series in the presence of 5 and 30% blood serum. The resulting apparent dissociation constants were determined to be K d =6±0.4 and 50±7 μM, respectively ( Fig. 4b ). Both experiments were fitted using a cooperativity of 1.5. To understand the cause of this strong shift in affinity, we analysed the effect of the most abundant blood protein, human serum albumin (HSA), on the binding of quercetin to PKA. Owing to its hydrophobic binding pockets, this protein is a universal transport protein for a wide range of molecules and is known to bind, among others, to flavonoids such as quercetin [20] . If adsorption of quercetin to a blood protein occurs, the free concentration of the small molecule available for a binding to PKA is reduced, resulting in a shift of the apparent binding constant. To test whether HSA can cause the observed shift in the apparent affinity of PKA to quercetin, we analysed the binding of quercetin to HSA ( Fig. 4c ). HSA was labelled with a fluorescent dye, and a titration series of quercetin was prepared (0.5 to 90 μM). The thermophoretic depletion showed a sigmoidal binding curve, which was best fitted using Hill's equation. From the data, we inferred a dissociation coefficient of 9.3±0.5 μM with a Hill coefficient of h =2.75±0.2, which is in good agreement with literature values [20] . This experiment shows that quercetin binds to HSA and thus is expected to influence the apparent affinity of PKA for quercetin in human serum. To prove that the effect of the shifted affinities in human serum is due to the presence of HSA, we performed a PKA–quercetin binding experiment in 50 mM HEPES buffer and added HSA at concentrations corresponding to 5 and 30% human serum ( Fig. 4d ). At 32 μM HSA, which corresponds to 5% human serum, we observed a K d =7.8±0.6 μM. At 190 μM HSA, which is the equivalent of 30% human serum, we measured a K d =43±6 μM. The observed shift in the apparent dissociation constant differed only by about 20% from those obtained in serum. As in these experiments buffer, ionic strength and viscosity were constant, the reduced apparent affinity in serum is most likely a result of the binding of quercetin to HSA. This ability of MST to quantify binding near in vivo conditions is of high importance as MST can resolve either shifted affinities or competing interactions in biological matrices. This is of importance as information on adverse binding behaviour is typically obtained through clinical studies involving intense efforts and the risk of possible harm for the volunteers. Today, most antibody affinities are determined by surface-based methods such as surface plasmon resonance [21] , [22] . This technique requires the immobilization of either the antigen or the antibody on a solid surface, potentially raising issues of steric hindrance or molecular activity. Even though surface-based methods are very sensitive, high-affinity interactions are often not accessible for measurement owing to mass transport effects, and transient binders are in most cases difficult to quantify [23] . To analyse interactions in the solution phase, techniques such as fluorescence correlation spectroscopy (FCS) [24] , back-scattering interferometry [25] , [26] , [27] and isothermal titration calorimetry [28] are often used. FCS is based on highly sensitive fluorescence microscopy, but relies on a significant change in the diffusion constant upon binding [24] . For this reason, FCS is only applicable to a limited number of biomolecular interactions. The other two methods are label-free and allow monitoring of interactions without disturbance by a label or surfacing; however, these techniques still suffer from limitations. Isothermal titration calorimetry, for example, has a low throughput and exceptionally high sample consumption. Back-scattering interferometry typically suffers from a refractive index background arising from a non-reacted ligand, particularly at high concentrations. In addition, temperature-induced changes of the refractive index may interfere with the binding signal and render the interpretation difficult. The results we presented suggest that MST is suitable for the quantification of protein–protein affinities and low-molecular-weight binders. Both are of great importance in current basic and pharmaceutical research. Interactions between two proteins of approximately the same molecular weight can be analysed with the same sensitivity as interactions of small molecules or even ions. We attribute this broad range of detectable binding events to the fact that thermophoresis is highly sensitive to changes in the size, charge and hydration shell of molecules. Furthermore, we demonstrate that interaction measurements can be performed in complex biological liquids. Such biological matrices have a strong influence on the binding behaviour. Their analysis provides additional information on the properties and efficacies of the molecules within the human body. Additional work is required to understand the intricacies of MST in more detail. Future work will show how exactly the amplitude of the MST signal reflects changes in the protein conformation or in its hydration shell (for example, release of water molecules from binding sites). The amplitude could give additional information on the binding location of the small molecule and, for example, could detect binding of a small molecule to a deep hydrophobic binding pocket or to the protein surface. In addition, we envisage label-free approaches using the intrinsic fluorescence of proteins in the ultraviolet regime to avoid possible effects of the fluorescent label on the binding. However, label-free approaches will complicate measurements in biological liquids owing to their inherent background signals. In conclusion, we show that MST provides a fast analysis of interactions with low sample consumption. The measurements equally cover highly affine interactions, as well as interactions of low affinity. We analysed the binding of a broad variety of biologically relevant proteins and found a good signal-to-noise ratio, even for binders that have a low molecular weight. Additionally, the quantification of binding works equally well in biological liquids, where considerable shifts towards lower effective affinities are found. Such information is crucial for studying biomolecule interactions in biology and in drug development. Theoretical background of thermophoresis When an aqueous solution is heated locally, molecules start moving along the temperature gradient. This molecular flow is opposed by mass diffusion. In the steady state, both effects balance, resulting in a stationary spatial concentration distribution [29] , [30] : The relative concentration depends solely on Soret coefficient S T of the molecule and the temperature rise Δ T=T – T 0 at the respective position. Soret coefficient is a measure of the strength of the thermophoretic molecule flow compared with ordinary diffusion. Although the theory of thermophoresis is still under debate, all theoretical descriptions agree that the molecular size and various surface parameters, such as charge and hydrophobicity, have an influence on Soret coefficient S T . Recent theoretical approaches also include the influence of the Seebeck effect: ions in the buffer move along a thermal gradient and give rise to an electric field, which in turn moves the molecules by electrophoresis [31] , [32] , [33] . As the buffer systems throughout this work used NaCl to set the ionic strength, the resulting Seebeck contribution was suggested to be small [33] . To illustrate the influence of biomolecular parameters on the thermophoretic effect, we have chosen a local thermodynamic description [7] . Experiments suggest that the Soret coefficient can be expressed by [34] with A being the molecule's surface area, σ eff the effective charge and Δ s hyd the hydration entropy of the molecule–solution interface . In addition, Soret coefficient depends on the Debye–Hueckel screening length λ DH , the dielectric constant ɛ and its temperature derivative β . As a result, thermophoresis is a measure for the state of a protein, and on binding we expect a change in the thermophoretic signal. A protein–protein interaction, for example, may change the surface area A , the hydration entropy Δ s hyd and the effective charge σ eff , whereas an ion binding to a protein will mainly affect the effective charge. The binding of an uncharged small molecule may change the hydration entropy, as water molecules on the protein surface are released or rearranged. It has already been shown that small conformational changes can affect several of the above parameters. Of note, any change in the thermophoretic parameters on binding allows MST to quantify a binding affinity. Fluorescence imaging and bleaching correction We used a Zeiss AxioScope A1 Vario microscope with a 40× Plan Fluar oil objective (Numerical aperture NA=1.3, Zeiss), excited with Luxeon high-power LEDs (cyan, red). The LEDs were built into a standard halogen lamp housing and driven at a current of 10–200 mA by an ILX Lightwave LD-3565 constant current source, providing low illumination noise levels. Fluorescence filters were from AHF-Analysentechnik for HEX (F36-542) and AlexaFluor647 (F36-523). Detection was provided with a 12-bit PCO Sensicam uv camera (PCO AG) with a pixel size of 8 μm×8 μm, a maximum quantum efficiency of 65%, and typically 8×8 pixel binning. Exposure times ranged between 100 and 500 ms. Infrared laser heating Temperature gradients were created with an infrared laser diode (Furukawa FOL1405-RTV-617-1480, 1480 nm, 320 mW maximum power) purchased from AMS Technologies AG. The infrared-laser beam couples into the path of light with a dichroic mirror (NT46-386) from Edmund Optics and is focused into the fluid with the microscope objective also used for fluorescence imaging. Typically, the temperature in the solution was raised by 5 K in the beam center, with a 1/ e 2 diameter of 25 μm. All measurements were performed at a room temperature of approximately 20 °C, except for the binding of hIFN-γ, which was performed at 5 °C to avoid proteolysis. Microfluidic chambers We used fused silica capillaries (Polymicro Technologies) with an inner diameter of about 100 μm and an outer diameter of 370 μm. Inner dimensions varied only by ±0.5 μm per 10 m capillary length. The well-defined thickness allowed for good control and repeatability of the temperature. Binding of molecules to the capillary surface was low and was tested by measuring residual fluorescence after rinsing the capillary with buffer. The sample volume was about 500 nl. Data analysis The change in concentration was averaged over a rectangular region around the center of heating. We corrected the fluorescence signal for the temperature dependency of the fluorescence emission [35] . Generally, the fluorescence was independent of the binding state. This correction did not include possible binding-dependent changes in the temperature response of the molecule. Slow conformational variations were recently reported by Ebbinghaus et al . [36] and can lead to an uncertainty when determining the exact depletion, but does not effect the precision of the analysis. The relative change in concentration was normalized to the saturation value, at which all molecules were in the bound state. The binding of ligands to a specific receptor is characterized by K d and the total concentration of binding sites, [B 0 ]. The determination of these two parameters can be achieved using saturation-binding curves obtained at equilibrium [37] . [L 0 ] equals the amount of added ligand at each data point and [BL] is the concentration of formed complexes between the binding sites, [B], and the ligand, [L]. The fitting function is derived from the law of mass action: For reactions with more than one ligand binding to one binding partner or in case of cooperativity on binding, the data were fitted using Hill's equation: with h being Hill coefficient, K d the dissociation constant and [L] the concentration of ligand. Equation (5) was only used when the free concentration of the ligand was not altered by the formation of the complex and [L]=[L 0 ] was approximately true. Proteins hIFN-γ (product PHP050) and its anti-IFN-γ antibody (product HCA043) were gifts from AbD Serotec. The antibody is a bivalent human recombinant Fab selected from the HuCAL GOLD phage display library and dimerized via a helix–turn–helix motif. The antibody was labelled with AlexaFluor 647 (Invitrogen) and used at a constant antibody concentration of 5 nM. Human IFN-γ was titrated from 0.1 to 700 nM. The experiments were performed in a standard PBS (1× PBS) solution. To prevent proteolysis, measurements in either buffer or E . coli extract were performed at 5 °C. The buffer conditions were 1× PBS with 5% bovine serum albumin and 0.01% Tween20. Before the measurement, samples were incubated for 1 h on ice. Chromotek GmbH provided the GFP, GBP, GBP mutant (GBP R37A) and RBP. GFP is a 28-kDa protein with intrinsic fluorescence. The GBP is a small 14.1-kDa protein originally isolated from the lymphocytes of a Llama Alpaca (Llama Pacos) immunized with purified GFP [12] . RBP is an RFP-binding protein with a molecular weight of 15 kDa and was used as a negative control. The measurements were performed in 1× PBS using 40 nM GFP and by titrating from 0.1 nM to 4 μM of GBP. CaM was purchased from AbD Serotec and labelled with AlexaFluor 647. The analysis was performed in 1× PBS. All CaM solutions contained a small amount of EDTA to bind any free Ca 2+ ions before mixing with the desired concentration of calcium ions. For the interaction analysis in serum, Crelux GmbH provided the protein kinase A and the inhibitor quercetin. The kinase was labelled with AlexaFluor 647 and was used at a final concentration of 300 nM. The binding was measured in 50 mM HEPES at pH 7.5 containing 100 mM NaCl and 5% DMSO. Quercetin was titrated from 11.5 nM to 50 μM, close to the solubility limit of the substance. After mixing the protein with quercetin, the serum was added and incubated for 1 h at room temperature. For the analysis of HSA with quercetin, HSA was labelled with AlexaFluor 647 and used at a final concentration of 50 nM. The titration series of quercetin ranged from 0.5 to 90 μM. The interaction was analysed in 50 mM HEPES buffer at pH 7.5 containing 100 mM NaCl. Labelling procedure The labelling was performed with reactive dyes using N-Hydroxysuccinimide (NHS)–ester chemistry, which reacts efficiently with the primary amines of proteins to form highly stable dye–protein conjugates. The labelling step requires that the protein be dissolved in a suitable labelling buffer at the correct pH. For protein labelling, the protein concentration was adjusted to 2–20 μM using the labelling buffer. Lower concentrations may result in loss of coupling efficiency. The solid fluorescent dye was dissolved in 100% DMSO at a concentration of about 1.3 mM and mixed thoroughly. Before mixing the protein and the dye, the concentration of the dye was adjusted to 2–3-fold concentration of the protein using the labelling buffer. Then, the protein and the fluorescent dye solutions were mixed in 1:1 ratio and incubated for 30 min at room temperature in the dark. Unreacted 'free' dye was eliminated by gelfiltration columns (Sephadex G25, GE Healthcare). The purity was monitored by measuring the ratio of protein to dye (for example, spectroscopically by measuring absorption at 280 nm for protein and 650 nm for the dye; molar absorbance: 250,000 M −1 cm −1 ) after the clean-up procedure. How to cite this article: Wienken, C. J. et al . Protein binding assays in biological liquids using microscale thermophoresis. Nat. Commun. 1:100 doi: 10.1038/ncomms1093 (2010).